CUL4 forms an E3 ligase with COP1 and SPA to promote light-induced degradation of PIF1 Plants undergo contrasting developmental programs in dark and light. Photomorphogenesis, a light-adapted programme is repressed in the dark by the synergistic actions of CUL4 COP1–SPA E3 ubiquitin ligase and a subset of basic helix-loop-helix transcription factors called phytochrome interacting factors (PIFs). To promote photomorphogenesis, light activates the phytochrome family of sensory photoreceptors, which inhibits these repressors by poorly understood mechanisms. Here, we show that the CUL4 COP1–SPA E3 ubiquitin ligase is necessary for the light-induced degradation of PIF1 in Arabidopsis . The light-induced ubiquitylation and subsequent degradation of PIF1 is reduced in the cop1 , spaQ and cul4 backgrounds. COP1, SPA1 and CUL4 preferentially form complexes with the phosphorylated forms of PIF1 in response to light. The cop1 and spaQ seeds display strong hyposensitive response to far-red light-mediated seed germination and light-regulated gene expression. These data show a mechanism by which an E3 ligase attenuates its activity by degrading its cofactor in response to light. Terrestrial flowering plants use dual developmental programmes early in their life cycle: skotomorphogenesis where postgerminative seedlings grow rapidly to emerge from subterranean darkness, and photomorphogenesis where rapid growth by elongation is inhibited to allow seedling body pattern formation suited to assemble photosynthetic apparatus for maximal light capture and autotrophic growth. Plants use multiple repressors of photomorphogenesis to prevent precocious germination and seedling emergence in the dark. These include 11 loci in Arabidopsis encoding CONSTITUTIVE PHOTOMORPHOGENIC/DEETIOLATED/FUSCA (COP/DET/FUS) genes and seven basic helix-loop-helix loci encoding phytochrome interacting factors (PIF1, PIF3-8; refs 1 , 2 , 3 ). These repressors fine tune seed germination and seedling development during the dark to light transition when young seedlings are especially vulnerable to toxicity of light exposure [1] , [2] , [3] . Among the repressors of photomorphogenesis, COP1 is a RING type E3 ubiquitin ligase that is evolutionarily conserved in many higher eukaryotes [4] . COP1 forms multiple complexes with SUPPRESSOR OF PHYA-105 (SPA1-4) family members [5] . These complexes, either by themselves or by forming CUL4 COP1–SPA E3 ubiquitin ligases, degrade the positively acting transcription factors through the ubiquitin proteasome system (UPS) to repress photomorphogenesis in the dark [6] . Strikingly, PIF1 directly interacts with COP1 and SPA complex and acts as a cofactor of COP1 E3 ubiquitin ligase to synergistically degrade the positively acting factor HY5 to repress photomorphogenesis in the dark [7] . PIFs also interact with DET1 and synergistically repress photomorphogenesis in the dark [8] . Therefore, the COP/DET/SPA and PIF complexes act independently as well as synergistically to prevent seed germination and seedling emergence in the dark. Under light, the phytochrome family of sensory photoreceptors perceives light signals and undergoes allosteric changes in structure from an inactive Pr form to a biologically active Pfr form [9] . The active Pfr forms of phytochromes translocate into nucleus [10] , and inhibit the repressors of photomorphogenesis by distinct mechanisms. For COP1, phytochromes induce a rapid reorganization of the COP1–SPA complex to reduce the function of COP1 and thereby stabilize the positively acting factors [11] . In addition, phytochromes promote nuclear exclusion of COP1 under light and thereby stabilizing the positive regulators of photomorphogenesis [12] , [13] . By contrast, the light-activated forms of phytochromes directly interact with PIFs and induce rapid phosphorylation, polyubiquitylation and UPS-mediated degradation of PIFs to promote photomorphogenesis [14] , [15] . The factors necessary for light-induced phosphorylation and polyubiquitylation of PIFs are under intense investigation. Recent data showed that direct physical interaction with phytochromes and rapid light-induced phosphorylation of PIFs are necessary for the UPS-mediated degradation [16] , [17] , [18] . Two kinases have been shown to phosphorylate PIFs in vitro [19] . For example, CK2 was shown to phosphorylate PIF1 in vitro [20] . A mutant form of PIF1 deficient in CK2 phosphorylation sites displayed reduced degradation in response to light in vivo , suggesting CK2 promotes PIF1 degradation. BIN2 phosphorylates PIF4 in vitro and BIN2-mediated phosphorylation affects degradation of PIF4 under light [21] . However, both CK2- and BIN2-mediated phosphorylation of PIFs are light independent, suggesting that additional kinases are necessary for light-induced phosphorylation of PIFs [22] . Recently, a CUL3 LRB E3 ubiquitin ligase was found to be necessary for the light-induced ubiquitylation and subsequent co-degradation of PIF3 and phyB under light [23] . However, the kinase and the E3 ubiquitin ligase necessary for the light-induced degradation of PIF1 are still unknown. Here, we show that the CUL4 COP1–SPA complex is necessary for the rapid light-induced degradation of PIF1. Moreover, contrary to their established role as repressors, our data show that COP1 and SPA proteins also function positively to promote seed germination in response to light. COP1 and SPA complex with CUL4 promote degradation of PIF1 Because PIF1 formed a complex with COP1 and SPA1, components of the E3 ubiquitin ligases in the dark [7] , we examined whether the CUL4 COP1–SPA E3 ubiquitin ligases also play a role in the light-induced degradation of PIF1 in Arabidopsis . We performed immunoblots for PIF1 levels in the individual components of the CUL4 COP1–SPA complex mutants both in the dark and light. Strikingly, the data show that the light-induced degradation of PIF1 is reduced in the cop1-4 , cop1-6 , spaQ and cul4cs ( CUL4 co-suppression) seedlings compared with wild type ( Fig. 1a–d ). PIF1 is also slightly more stable in cul4-1 , a weak allele of cul4 compared with wild-type seedlings under light ( Supplementary Fig. 1 ). Among all these mutants, both spaQ and cul4cs displayed the slowest rate of degradation of PIF1. PIF1 is more abundant both in the dark and light in spaQ and cul4cs compared with wild type, indicating that SPA and CUL4 are involved in PIF1 degradation both in the dark and light. The increased abundance of PIF1 in these mutants is at the post-translational level as PIF1 mRNA in these mutants is similar to wild type ( Supplementary Fig. 2 ). Moreover, this early degradation is regulated by phyA as it is eliminated in the phyA background ( Supplementary Fig. 3 ). The phyB plays a minor role under these conditions ( Supplementary Fig. 3 ) [17] . To identify which SPA protein is necessary for this response, we performed immunoblots for PIF1 levels in spa1, spa2, spa12, spa123 and spa124 mutants compared with wild type. Results show that the SPA family members redundantly regulate the light-induced degradation of PIF1 ( Supplementary Fig. 4 ). The above experiments were performed to examine PIF1 stability at early times immediately after exposure to small amount of light pulses. To examine PIF1 stability under prolonged light conditions, we performed immunoblots using the above mutants under continuous red light. Strikingly, the data show that PIF1 is degraded in the cop1-4 and cul4cs backgrounds similar to wild type ( Supplementary Fig. 5 ). PIF1 is also degraded in the spaQ background under these conditions; however, the rate of degradation is much slower in the spaQ compared with other mutants ( Supplementary Fig. 5 ). These data suggest that the CUL4 COP1–SPA E3 ubiquitin ligase regulates PIF1 levels during dark to light transition. However, additional E3 ubiquitin ligase(s) regulate PIF1 level under prolonged light conditions. 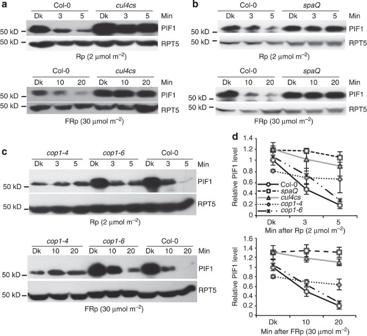Figure 1: COP1 and SPA complex with CUL4 promote degradation of PIF1. Immunoblots showing reduced degradation of native PIF1 in thecul4cs(a),spaQ(b),cop1-4andcop1-6(c) backgrounds in response to red and far-red light compared with wild-type seedlings. Four-day-old dark-grown seedlings were either kept in darkness or exposed to a pulse of red or far-red light and then incubated in the dark for the duration indicated before being sampled for protein extraction. Total protein (∼30 μg) was separated on an 8% SDS–PAGE gel, transferred to PVDF membrane and probed with anti-PIF1 and anti-RPT5 antibodies. (d) Quantification of PIF1 degradation kinetics in response to red and far-red light is shown. RPT5 was used for normalization. The error bars indicate s.e.m. (n=3). Figure 1: COP1 and SPA complex with CUL4 promote degradation of PIF1. Immunoblots showing reduced degradation of native PIF1 in the cul4cs ( a ), spaQ ( b ), cop1-4 and cop1-6 ( c ) backgrounds in response to red and far-red light compared with wild-type seedlings. Four-day-old dark-grown seedlings were either kept in darkness or exposed to a pulse of red or far-red light and then incubated in the dark for the duration indicated before being sampled for protein extraction. Total protein ( ∼ 30 μg) was separated on an 8% SDS–PAGE gel, transferred to PVDF membrane and probed with anti-PIF1 and anti-RPT5 antibodies. ( d ) Quantification of PIF1 degradation kinetics in response to red and far-red light is shown. RPT5 was used for normalization. The error bars indicate s.e.m. ( n =3). Full size image Recently, a CUL3 LRB E3 ubiquitin ligase has been shown to be necessary for the light-induced co-degradation of PIF3 and phyB [23] . To examine whether PIF1 is also degraded through other Cullins, we performed immunoblots for PIF1 levels in cul1 and cul3 mutants. Results show that PIF1 is largely degraded in the cul1-6 , cul3a , cul3b and cul3ab double-mutant backgrounds similar to wild type ( Supplementary Fig. 6 ). In addition, the light-induced degradation of phyA is unaffected in the cul4cs , cop1 , spaQ backgrounds ( Supplementary Fig. 7 ). These data suggest that, unlike PIF3 and phyB [23] , PIF1 and phyA may not be co-degraded through the CUL4 COP1–SPA E3 ubiquitin ligase complexes. CUL4 based E3 ligase promote ubiquitylation of PIF1 The light-induced degradation of PIFs is UPS-mediated and involves phosphorylation and polyubiquitylation of PIFs [16] , [17] , [20] , [23] . We examined whether the phosphorylation or ubiquitylation of PIF1 is affected in the cop1-4 , spaQ and cul4cs seedlings. The data show that the light-induced ubiquitylation of TAP-PIF1 is strongly reduced in all three backgrounds compared with wild type with the strongest effect in the spaQ ( Fig. 2a–c ). This is consistent with the degradation rate in the spaQ background. The data also show that the light-induced phosphorylation is unaffected in these backgrounds, suggesting that these factors are involved in polyubiquitylation of PIF1 in response to light. 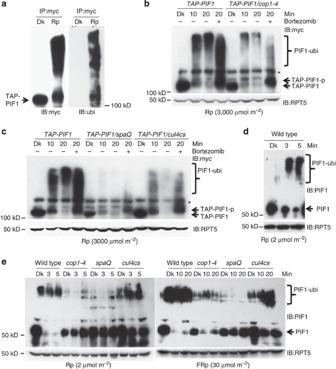Figure 2: COP1 and SPA complex with CUL4 promote ubiquitylation of PIF1. (a) PIF1 is ubiquitylated in response to light. TAP-PIF1 was immunoprecipitated using anti-myc antibody from dark and light exposed seedlings and probed with anti-myc (left) or anti-ubi (right) antibodies. (b,c) Ubiquitylated PIF1 is less abundant in thecop1-4(b),spaQandcul4cs(c) backgrounds in response to light. Four-day-old dark-grown seedlings were either kept in darkness or exposed to a pulse of red light and then incubated in the dark for the duration indicated before being sampled for protein extraction. One batch of seedlings was pretreated with the proteasome inhibitor (40 μM Bortezomib) before being exposed to red light. Total protein (∼30 μg) was separated on a 6.5% SDS–PAGE gel, transferred to PVDF membrane and probed with anti-myc and anti-RPT5 antibodies. The ubiquitylated bands, TAP-PIF1 and phosphorylated form of TAP-PIF1 are indicated. *, indicates a cross-reacting band. (d) Native PIF1 is not ubiquitylated in darkness under true dark condition. Col-0 seeds were stratified at 4 °C for 5 days followed by 5 min of FR light (34 μmol m−2s−1) and then kept in darkness for 4 days at 21 °C. Seedlings were either kept in darkness or exposed to 2 μmol m−2of red light pulse followed by 3 and 5 min incubation in darkness. Total protein (∼30 μg) was separated on an 8% SDS–PAGE gel, transferred to PVDF membrane and probed with anti-PIF1 and anti-RPT5 antibodies. (e) The light-induced ubiquitylation of native PIF1 is reduced incop1-4andspaQcompared with wild-type seedlings. Immunoblots showing ubiquitylation and subsequent degradation of native PIF1 incop1-4andspaQbackgrounds in response to red (left) and far-red light (right) compared with wild type. Four-day-old dark-grown seedlings were either kept in darkness or exposed to a pulse of red or far-red light and then incubated in the dark for the duration indicated before being sampled for protein extraction. Total protein (∼30 μg) was separated on an 8% SDS–PAGE gel, transferred to PVDF membrane and probed with anti-PIF1 and anti-RPT5 antibodies. Figure 2: COP1 and SPA complex with CUL4 promote ubiquitylation of PIF1. ( a ) PIF1 is ubiquitylated in response to light. TAP-PIF1 was immunoprecipitated using anti-myc antibody from dark and light exposed seedlings and probed with anti-myc (left) or anti-ubi (right) antibodies. ( b , c ) Ubiquitylated PIF1 is less abundant in the cop1-4 ( b ), spaQ and cul4cs ( c ) backgrounds in response to light. Four-day-old dark-grown seedlings were either kept in darkness or exposed to a pulse of red light and then incubated in the dark for the duration indicated before being sampled for protein extraction. One batch of seedlings was pretreated with the proteasome inhibitor (40 μM Bortezomib) before being exposed to red light. Total protein ( ∼ 30 μg) was separated on a 6.5% SDS–PAGE gel, transferred to PVDF membrane and probed with anti-myc and anti-RPT5 antibodies. The ubiquitylated bands, TAP-PIF1 and phosphorylated form of TAP-PIF1 are indicated. *, indicates a cross-reacting band. ( d ) Native PIF1 is not ubiquitylated in darkness under true dark condition. Col-0 seeds were stratified at 4 °C for 5 days followed by 5 min of FR light (34 μmol m −2 s −1 ) and then kept in darkness for 4 days at 21 °C. Seedlings were either kept in darkness or exposed to 2 μmol m −2 of red light pulse followed by 3 and 5 min incubation in darkness. Total protein ( ∼ 30 μg) was separated on an 8% SDS–PAGE gel, transferred to PVDF membrane and probed with anti-PIF1 and anti-RPT5 antibodies. ( e ) The light-induced ubiquitylation of native PIF1 is reduced in cop1-4 and spaQ compared with wild-type seedlings. Immunoblots showing ubiquitylation and subsequent degradation of native PIF1 in cop1-4 and spaQ backgrounds in response to red (left) and far-red light (right) compared with wild type. Four-day-old dark-grown seedlings were either kept in darkness or exposed to a pulse of red or far-red light and then incubated in the dark for the duration indicated before being sampled for protein extraction. Total protein ( ∼ 30 μg) was separated on an 8% SDS–PAGE gel, transferred to PVDF membrane and probed with anti-PIF1 and anti-RPT5 antibodies. Full size image To examine the light-induced ubiquitylation of native PIF1, we performed western blots on protein extracts from wild-type, cop1-4 , spaQ and cul4cs seedlings with anti-PIF1 antibody. Results show that the ubiquitylation of native PIF1 is strongly reduced in cop1-4 and spaQ mutants compared with wild type under both red and far-red light conditions ( Fig. 2e ). PIF1 is ubiquitylated in the wild-type and cul4cs backgrounds both in the dark and light exposure. However, light signals induced additional slow mobility bands in the wild-type background. These data are inconsistent with the TAP-PIF1 ubiquitylation as shown above, which did not display any ubiquitylation in the dark. This difference is most likely due to the strong sensitivity of native PIF1 to light exposure as the degradation rate of native PIF1 is much faster than that of TAP-PIF1 (ref. 17 ). Moreover, these experiments were performed under standard seedling growth conditions where seeds are plated in white light and exposed to prolonged saturated white light for inducing complete germination. To examine whether native PIF1 is ubiquitylated in the dark, we grew wild-type seedlings under true dark conditions as previously described [24] , and performed western blots for native PIF1. Results show that the native PIF1 is not ubiquitylated in the dark if the seedlings were grown under true dark conditions ( Fig. 2d ). However, red light exposure strongly induced ubiquitylation of native PIF1. Taken together, these data strongly suggest that COP1 and SPA proteins are necessary for the light-induced polyubiquitylation of PIF1. COP1 and SPA complex with CUL4 directly interact with PIF1 If PIF1 is degraded through the CUL4 COP1–SPA complex, PIF1 is expected to associate with these proteins i n vivo . Recently, we have shown that PIF1 interacts with COP1 and SPA1 in the dark. Moreover, the APB domain of PIF1 interacts with the WD40 domain of COP1 (ref. 7 ). We performed yeast two-hybrid assays using the full-length and various deletion fragments of PIF1 and SPA1. Results show that the APA domain of PIF1 is necessary for the interaction with the WD40 domain of SPA1 ( Supplementary Fig. 8a-c ). Moreover, PIF1 interacted with both COP1 and SPA1 in an in vitro interaction assays ( Supplementary Fig. 9 ). To examine the light-dependent interaction among these proteins, we performed in vivo co-immunoprecipitation assays using transgenic plants expressing both proteins. Results show that PIF1 strongly interacts with SPA1, COP1 and CUL4 in a light-dependent manner ( Fig. 3a–c ). PIF1 also displayed interaction with COP1 in the dark as previously shown [7] . However, these assays showed that CUL4, COP1 and SPA1 interacted preferentially with a slow migrating form of PIF1 in response to light ( Fig. 3a–d ). The slow migrating form of PIF1 has previously been shown as the phosphorylated forms of PIF1 (ref. 17 ). These data suggest that COP1–SPA complexes preferentially recruit the phosphorylated forms of PIF1 in the CUL4 COP1–SPA E3 ubiquitin ligase for ubiquitylation and subsequent degradation in response to light. 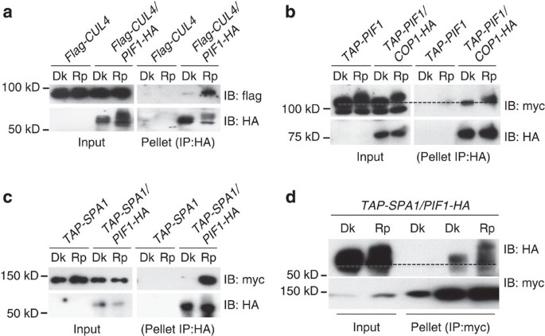Figure 3: COP1 and SPA complex with CUL4 directly interact with PIF1. (a) PIF1-HA interacts with Flag-CUL4 in anin vivoco-immunoprecipitation (co-IP) assay. The input and pellet fractions are indicated. Seedlings were pretreated with the proteasome inhibitor (40 μM bortezomib) for 5 h before being exposed to red light. Total protein was extracted from 4-day-old dark-grown seedlings either exposed to a pulse of red light (Rp; 3,000 μmol m−2) or kept in the dark (Dk). Co-IP was carried out using the anti-HA antibody and then probed with anti-flag and anti-HA antibodies. (b) TAP-PIF1 interacts with COP1-HA in response to light. The input and pellet fractions are indicated. Co-IP was carried out using the anti-HA antibody and then probed with anti-myc and anti-HA antibodies. (c) PIF1-HA interacts with TAP-SPA1in vivoin response to red light. The input and pellet fractions of thein vivoco-IP assay are indicated. Co-IP was carried out using the anti-HA antibody and then probed with anti-myc and anti-HA antibodies. (d) TAP-SPA1 interacts with both the phosphorylated and unphosphorylated forms of PIF1. The input and pellet fractions are indicated. Co-IP was carried out using the anti-myc antibody and then probed with anti-HA and anti-myc antibodies. Figure 3: COP1 and SPA complex with CUL4 directly interact with PIF1. ( a ) PIF1-HA interacts with Flag-CUL4 in an in vivo co-immunoprecipitation (co-IP) assay. The input and pellet fractions are indicated. Seedlings were pretreated with the proteasome inhibitor (40 μM bortezomib) for 5 h before being exposed to red light. Total protein was extracted from 4-day-old dark-grown seedlings either exposed to a pulse of red light (Rp; 3,000 μmol m −2 ) or kept in the dark (Dk). Co-IP was carried out using the anti-HA antibody and then probed with anti-flag and anti-HA antibodies. ( b ) TAP-PIF1 interacts with COP1-HA in response to light. The input and pellet fractions are indicated. Co-IP was carried out using the anti-HA antibody and then probed with anti-myc and anti-HA antibodies. ( c ) PIF1-HA interacts with TAP-SPA1 in vivo in response to red light. The input and pellet fractions of the in vivo co-IP assay are indicated. Co-IP was carried out using the anti-HA antibody and then probed with anti-myc and anti-HA antibodies. ( d ) TAP-SPA1 interacts with both the phosphorylated and unphosphorylated forms of PIF1. The input and pellet fractions are indicated. Co-IP was carried out using the anti-myc antibody and then probed with anti-HA and anti-myc antibodies. Full size image COP1 and SPA promote seed germination in response to light To examine the biological significance of this rapid and transient light-induced degradation of PIF1, we examined photomorphogenic phenotypes in these mutants. Although, cop1 and spaQ seedlings display strong constitutively photomorphogenic phenotypes in the dark as previously described ( Supplementary Fig. 10 ; ref. 2 ), a positive role for cop1 in the light-induced cotyledon opening responses has been previously described [25] . Moreover, the cop1 , spaQ and cul4cs seeds do not germinate constitutively in the dark ( Fig. 4a,b ; ref. 7 ). Because of the transient and early phyA-mediated degradation of PIF1 as well as exclusive role of PIF1, we focused on seed germination, a more light-sensitive response, under far-red and red light [26] , [27] . Strikingly, cop1-4, cop1-6 and spaQ displayed strong hyposensitive response to far-red light-mediated seed germination ( Fig. 4a ). In addition, spaQ showed hyposensitive response to red light for seed germination assays ( Fig. 4b ). Genetic analyses also showed that pif1 is epistatic to cop1 and spaQ under both far-red and red light conditions ( Fig. 4c ), suggesting that PIF1 functions downstream of COP1 and SPA proteins in regulating seed germination. 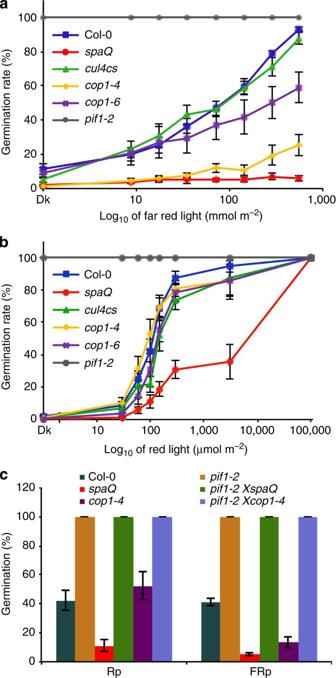Figure 4:cop1andspaQdisplay hyposensitive phenotype for seed germination. (a) Fluence rate response curves showing hyposensitive phenotypes of thecop1-4, cop1-6andspaQcompared with wild-type under far-red light. Seed germination assays were performed as previously described26,39. Briefly, same-age seeds of all genotypes were surface sterilized within 1 h of imbibition and plated on MS plates (0.1 g l−1MS salt), exposed to 5 min of FR light (34 μmol m−2s−1) before being kept in the dark for 48 h at 21 °C. The seeds were then exposed to an increasing amount of far-red light as indicated. Plates were wrapped in aluminium foil at 21 °C for 6 additional days in the dark before being scored. The error bars indicate s.e.m. (n=3). (b) ThespaQseeds require a higher amount of red light for completion of germination than the wild-type seeds. Red light-mediated seed germination assay was performed as described26,39. Briefly, same-age seeds of all genotypes were surface sterilized within 1 h of imbibition, exposed to 5 min of FR light (34 μmol m−2s−1) before being exposed to an increasing amount of red light as indicated. Plates were wrapped in aluminium foil at 21 °C for 6 days in the dark before being scored. The error bars indicate sem (n=3). (c)pif1is epistatic tocop1andspaQin seed germination assays. Bar graph shows the percentage of seed germination of various genotypes at two different conditions: 100 μmol m−2red (Rp) light and 71 mmol m−2far red (FRp) light. Seed germination assays were performed as described above. The error bars indicate s.e.m. (n=3). Figure 4: cop1 and spaQ display hyposensitive phenotype for seed germination. ( a ) Fluence rate response curves showing hyposensitive phenotypes of the cop1-4, cop1-6 and spaQ compared with wild-type under far-red light. Seed germination assays were performed as previously described [26] , [39] . Briefly, same-age seeds of all genotypes were surface sterilized within 1 h of imbibition and plated on MS plates (0.1 g l −1 MS salt), exposed to 5 min of FR light (34 μmol m −2 s −1 ) before being kept in the dark for 48 h at 21 °C. The seeds were then exposed to an increasing amount of far-red light as indicated. Plates were wrapped in aluminium foil at 21 °C for 6 additional days in the dark before being scored. The error bars indicate s.e.m. ( n =3). ( b ) The spaQ seeds require a higher amount of red light for completion of germination than the wild-type seeds. Red light-mediated seed germination assay was performed as described [26] , [39] . Briefly, same-age seeds of all genotypes were surface sterilized within 1 h of imbibition, exposed to 5 min of FR light (34 μmol m −2 s −1 ) before being exposed to an increasing amount of red light as indicated. Plates were wrapped in aluminium foil at 21 °C for 6 days in the dark before being scored. The error bars indicate sem ( n =3). ( c ) pif1 is epistatic to cop1 and spaQ in seed germination assays. Bar graph shows the percentage of seed germination of various genotypes at two different conditions: 100 μmol m −2 red (Rp) light and 71 mmol m −2 far red (FRp) light. Seed germination assays were performed as described above. The error bars indicate s.e.m. ( n =3). Full size image Degradation of PIF1 is reduced in cop1-4 and spaQ seeds Because PIF1 has an exclusive role in seed germination [26] , and cop1-4 and spaQ displayed defects in seed germination in response to light ( Fig. 4 ), we examined PIF1 levels in the wild type and these two mutant seeds under dark and light exposure. Results show that the light-induced degradation of native PIF1 is strongly reduced in cop1-4 and is completely absent in the spaQ compared with wild-type seeds ( Fig. 5a,b ). To examine whether gene expression is altered in these backgrounds, we performed quantitative PCR with reverse transcription (qRT–PCR) analyses of a few PIF1 target genes at the seed stage under far-red light. Results show that the expression of the PIF1 target genes under far-red light is increased in these mutants compared with wild-type seeds, consistent with the PIF1 level in these backgrounds ( Fig. 5c ). These data suggest that COP1 and SPA proteins promote seed germination by inducing degradation of PIF1 in response to red and far-red light. 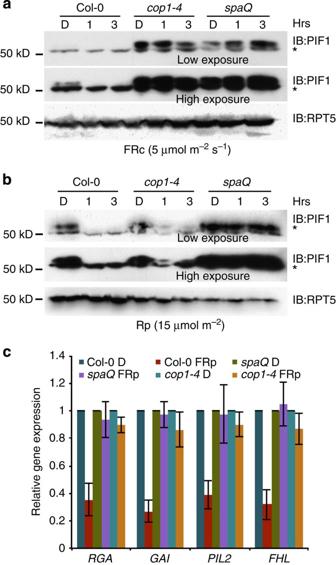Figure 5: Light-induced degradation of PIF1 is reduced incop1-4andspaQseeds. (a,b) Light-induced degradation of native PIF1 is reduced incop1-4andspaQmutants compared with wild-type seeds under far-red (a) and red (b) light. Seeds (0.02 g) of all genotypes were surface sterilized within 1 h of imbibition and plated on MS plates (0.1 g l−1MS salt) with filter paper, exposed to 15 min of FR light (3.2 μmol m−2s−1). For red light, these plates were kept in the dark for 48 h and then either kept in darkness or exposed to a pulse of red light (15 μmol m−2) before being stored in darkness for the duration indicated. For far-red light, these plates were kept in the dark for 48 h at 21 °C. The plates were then either kept in darkness or exposed to 5 μmol m−2s−1continuous far-red light for the duration indicated. Total protein was extracted from all the samples and separated on an 8% SDS–PAGE gel, transferred to PVDF membrane and probed with anti-PIF1 and anti-RPT5 antibodies. *, indicates cross-reacting band. (c) The expression of PIF1 target genes is increased incop1andspaQcompared with wild-type seeds under far-red light. Bar graph shows expression of various PIF1 target genes in the indicated genotypes in the dark and far-red light. Seeds of all genotypes were imbibed for 1 h on MS plates with 100 μM paclobutrazol, exposed to 5 min of FR light (34 μmol m−2s−1) and kept in the dark for 48 h. Total RNA was isolated from 48-h-old dark-grown seeds and 48-h-old dark-grown seeds exposed to far-red light (100 μmol m−2) for 1 h. The error bars indicate s.e.m. (n=3). Figure 5: Light-induced degradation of PIF1 is reduced in cop1-4 and spaQ seeds. ( a , b ) Light-induced degradation of native PIF1 is reduced in cop1-4 and spaQ mutants compared with wild-type seeds under far-red ( a ) and red ( b ) light. Seeds (0.02 g) of all genotypes were surface sterilized within 1 h of imbibition and plated on MS plates (0.1 g l −1 MS salt) with filter paper, exposed to 15 min of FR light (3.2 μmol m −2 s −1 ). For red light, these plates were kept in the dark for 48 h and then either kept in darkness or exposed to a pulse of red light (15 μmol m −2 ) before being stored in darkness for the duration indicated. For far-red light, these plates were kept in the dark for 48 h at 21 °C. The plates were then either kept in darkness or exposed to 5 μmol m −2 s −1 continuous far-red light for the duration indicated. Total protein was extracted from all the samples and separated on an 8% SDS–PAGE gel, transferred to PVDF membrane and probed with anti-PIF1 and anti-RPT5 antibodies. *, indicates cross-reacting band. ( c ) The expression of PIF1 target genes is increased in cop1 and spaQ compared with wild-type seeds under far-red light. Bar graph shows expression of various PIF1 target genes in the indicated genotypes in the dark and far-red light. Seeds of all genotypes were imbibed for 1 h on MS plates with 100 μM paclobutrazol, exposed to 5 min of FR light (34 μmol m −2 s −1 ) and kept in the dark for 48 h. Total RNA was isolated from 48-h-old dark-grown seeds and 48-h-old dark-grown seeds exposed to far-red light (100 μmol m −2 ) for 1 h. The error bars indicate s.e.m. ( n =3). Full size image As members of the bHLH family of transcription factors, PIFs have been shown to repress both molecular and morphological phenotypes in phytochrome signalling pathways [1] . However, the mechanisms by which phytochromes remove these repressors are beginning to be unravelled. The extensive biochemical and genetic evidence presented here strongly suggest that CUL4 COP1–SPA complex functions as an E3 ubiquitin ligase for the rapid light-induced degradation of PIF1. PIF1 is more abundant in cul4cs , cop1-4 and spaQ compared with wild-type backgrounds under light conditions ( Figs 1 and 5a,b ). The light-induced ubiquitylation of PIF1 is strongly reduced in these backgrounds compared with wild type ( Fig. 2 ). Moreover, PIF1 directly interacts with COP1 and SPA1 both in vitro and in yeast cells ( Supplementary Figs 8 and 9 ). PIF1 also forms complexes with CUL4, COP1 and SPA1 in vivo ( Fig. 3 ). Strikingly, CUL4, COP1 and SPA1 preferentially associated with the phosphorylated forms of PIF1 than the non-phosphorylated PIF1 under light exposure. Consistent with the above molecular evidence, cop1-4 and spaQ show a strong reduction in far-red and red light-induced seed germination and induction of PIF1 target gene expression ( Figs 4a,b and 5c ). Moreover, genetic evidence shows that PIF1 is epistatic to cop1-4 and spaQ in seed germination assays ( Fig. 4d ). Although, these data do not show that CUL4 COP1–SPA complex directly ubiquitylate PIF1 in vitro , the combined molecular, genetic and photobiological data presented here strongly suggest that the CUL4 COP1–SPA complex is involved in the light-induced ubiquitylation and subsequent degradation of PIF1. Previously, COP1 has been shown to directly ubiquitylate positively acting transcription factors and phytochromes in vitro [3] , [28] . In this process, PIFs and SPA proteins enhance the COP1 activity in vitro [7] , [28] , [29] , [30] . The enhancement of COP1 activity is also consistent with the synergistic stabilization of COP1 substrates (for example, HY5/HFR1/LAF1) and synergistic morphological phenotypes in the cop1spa1 versus cop1 and cop1pifQ versus cop1 mutants, respectively [7] , [28] , [29] , [30] . However, PIFs are not directly ubiquitylated by COP1 in vitro [7] , [28] . These data suggest a dichotomy for these E3 ubiquitin ligases, where COP1–SPA complexes can directly ubiquitylate the positively acting transcription factors (for example, HY5/LAF1/HFR1) in vitro , while the formation of the CUL4 COP1–SPA complex is necessary for the ubiquitylation of PIF1 and possibly other PIFs. Further biochemical characterizations are necessary to distinguish these possibilities. The availability of the two groups of substrates (PIFs and HY5/LAF1/HFR1) will help facilitate these studies. The relative abundance of PIF1 and PIF3 levels in cop1 and spa mutants also highlights the differences in the mechanisms of PIF regulation. PIF3 has been shown to be unstable in the cop1-4 and spa123 triple-mutant backgrounds in the dark [23] , [24] , [31] , suggesting that COP1 and SPA proteins are necessary for the stability of PIF3 in the dark. In contrast, while PIF1 level is also lower in cop1-4 compared with wild type, PIF1 is much more abundant in the spaQ mutants compared with wild type in the dark ( Fig. 1 ). PIF1 and PIF3-5 are stabilized by DET1 in the dark [8] . These data suggest that the CUL4 COP1–SPA E3 ubiquitin ligase is involved in PIF1 degradation under these conditions, and that different PIF family members are differentially regulated by different E3 ubiquitin ligases both in the dark and light conditions. Recently, a CUL3 LRB E3 ubiquitin ligase has been shown to directly ubiquitylate PIF3 in vitro , and is necessary for the light-induced co-degradation of PIF3 and phyB in vivo [23] . Examination of PIF1 level in cul3ab double mutant shows that CUL3 is not necessary for the light-induced degradation of PIF1 under these conditions ( Supplementary Fig. 6 ). PIF1 showed the highest affinity for phyA compared with other PIFs [32] . The phyA also plays a major role in degrading PIF1, whereas phyB plays a minor role under these conditions ( Supplementary Fig. 3 ) [17] . These data not only highlight the mechanistic details of PIF degradation, but also show the roles of different phytochromes under dark to light transition as well as under prolonged light conditions. In the dark, phyA is more abundant than other phytochromes [33] , and plays a major role in the light-induced transcriptional regulation under both red and far-red light conditions [34] . However, phyA is degraded through the UPS in response to red light [35] , whereas phyB plays a major role under prolonged red light conditions. Consistent with these data, the evidence presented here also suggest a division of labour for various E3 Ubiquitin ligases where CUL4 COP1–SPA complex plays a major role in phyA-mediated early light-induced degradation of PIF1, while CUL3 LRB complex plays a major role in phyB-mediated degradation of PIF3 and possibly other PIFs under prolonged light conditions. Additional kinetic analyses for the role of these E3 ligases in degrading multiple PIFs are necessary to draw a more robust conclusion. Collectively, the data presented here show a novel function of CUL4 COP1–SPA complex in promoting photomorphogenesis by acting as an E3 ubiquitin ligase for PIF1. In the dark, this E3 ubiquitin ligase degrades the positively acting transcription factors to prevent photomorphogenesis [3] . In this process, PIFs act as cofactors to enhance the substrate recruitment, auto- and trans-ubiquitylation of COP1 to synergistically repress photomorphogenesis in the dark [7] ( Fig. 6 , left). These two activities along with others establish a sufficiently repressed state to ensure prevention of precocious photomorphogenesis in the dark. However, immediately upon light exposure, the CUL4 COP1–SPA E3 ubiquitin ligase prevents over-repression of light responses by degrading its cofactor PIF1 to allow gradual initiation of photomorphogenesis ( Fig. 6 , right). These data highlight a novel signalling mechanism where an E3 ubiquitin ligase attenuates its activity by degrading its cofactor in response to light. 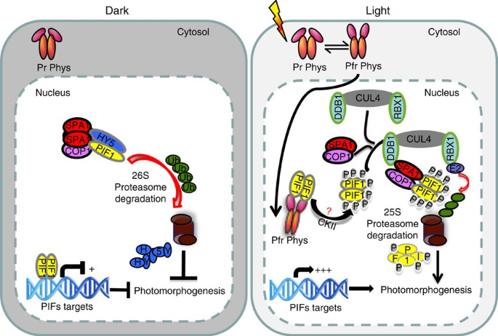Figure 6: A model showing light regulation of PIF1 during photomorphogenesis. Left, in the dark, the biologically inactive Pr form of phytochrome is localized in the cytosol. The nuclear localized PIF1 homodimers bind to the promoter region of light-regulated target genes and repress their expression to prevent photomorphogenesis. In addition, PIF1 interacts with the COP1–SPA1 E3 ubiquitin ligase complexes and enhances the E3 ligase activity for HY5 degradation. The dual functions of PIF1 ensure the synergistic inhibition of photomorphogenesis. Right, upon light exposure, the biologically active Pfr form of phytochrome translocates into nucleus. The interaction between Pfr phys and PIF1 triggers the rapid light-induced phosphorylation of PIF1 through an unknown kinase. The protein kinase CK2 also phosphorylates PIF1 and this phosphorylation is necessary for light-induced degradation. The phosphorylated form of PIF1 is then recruited to the CUL4COP1–SPA1complex for rapid ubiquitylation and subsequent degradation through the 26S proteasome pathway. The destruction of the negative regulator, PIF1, derepresses the light-regulated gene expression and thereby promotes photomorphogenesis. Figure 6: A model showing light regulation of PIF1 during photomorphogenesis. Left, in the dark, the biologically inactive Pr form of phytochrome is localized in the cytosol. The nuclear localized PIF1 homodimers bind to the promoter region of light-regulated target genes and repress their expression to prevent photomorphogenesis. In addition, PIF1 interacts with the COP1–SPA1 E3 ubiquitin ligase complexes and enhances the E3 ligase activity for HY5 degradation. The dual functions of PIF1 ensure the synergistic inhibition of photomorphogenesis. Right, upon light exposure, the biologically active Pfr form of phytochrome translocates into nucleus. The interaction between Pfr phys and PIF1 triggers the rapid light-induced phosphorylation of PIF1 through an unknown kinase. The protein kinase CK2 also phosphorylates PIF1 and this phosphorylation is necessary for light-induced degradation. The phosphorylated form of PIF1 is then recruited to the CUL4 COP1–SPA1 complex for rapid ubiquitylation and subsequent degradation through the 26S proteasome pathway. The destruction of the negative regulator, PIF1, derepresses the light-regulated gene expression and thereby promotes photomorphogenesis. Full size image Cellular signalling involves both positive and negative regulators to fine tune developmental programs. In most cases, this is achieved by using different factors acting positively or negatively in the pathway. Opposite roles of the same protein in a biological process have been described in association with other factors [36] , [37] . This is mostly common in transcription factors that recruit activator or repressor complexes to regulate gene expression [38] . Our data also provide a biochemical explanation for a novel signalling mechanism where a well-established master negative regulator complex acts positively to promote plant morphogenesis in response to light. Plant growth conditions and measurements Plants were grown in Metro-Mix 200 soil (Sun Gro Horticulture, Bellevue, WA, USA) under continuous light at 24±0.5 °C. Seeds were sterilized and plated on Murashige and Skoog (MS) growth medium containing 0.9% agar without sucrose as described [39] . The plates were kept at 4 °C in the dark for 3 to 4 days to stratify and then exposed to 3 h of white light at room temperature before being placed in the dark for 21 h. The plates were incubated at 21 °C for an additional 3 days in the dark or light as indicated. Arabidopsis thaliana wild type and various mutants ( pif1, cop1-4, cop1-6, spa1, spa2, spa12, spa123, spa124, spaQ, cul1-6, cul3a, cul3b, cul3ab, cul4-1 and cul4cs ) in the Col-0 background were used [6] , [32] , [40] , [41] , [42] , [43] , [44] , [45] , [46] , [47] , [48] . For generation of different spaQpif1 mutant, pif1 and spaQ were crossed to obtain the F1 seeds. The quintuple mutant was selected by genotyping and phenotypic characterization of the F2 population. The seed germination assay was performed as described [26] , [39] . Briefly, triplicates of 50 seeds for each genotype were surface sterilized and plated on MS medium (0.1 g l −1 MS salt) within 1 h of imbibition. For phyB-dependent seed germination, the plates were treated with either far-red light (34 μmol m −2 s −1 ) for 5 min or far-red followed by increasing amount of red light before being placed in the dark at 21 °C. Germination was scored after 6 days of growth. For phyA-dependent seed germination, plates were kept in the dark at 21 °C for 48 h after the 5-min treatment of far-red light (34 μmol m −2 s −1 ). The plates were then either kept in darkness or treated with increasing amount of far-red light and kept in the dark at 21 °C for an additional 4 days before being scored for germination. RNA extraction and qRT–PCR The qRT–PCR analysis was performed as described with minor variations [7] . Briefly, wild-type Col-0 and various mutant seeds were imbibed on MS plates containing 100 μM paclobutrazol for 1 h. The plates were treated with far-red light treatment (34 μmol m −2 s −1 ) for 5 min and kept in the dark at 21 °C for 48 h. Seed samples were either directly collected into liquid nitrogen (dark samples) or treated with 100 μmol m −2 FRp and collected after 1 h dark incubation (FRp samples). Total RNA from seeds was isolated using the Spectrum plant total RNA Kit (Sigma-Aldrich Co., St Louis, MO). Two micrograms RNA was treated with DNase I to eliminate genomic DNA and then reverse transcribed using Moloney murine leukaemia virus reverse transcriptase (Life Technologies Co., Carlsbad, CA) as per the manufacturer’s protocol. Power SYBR Green RT-PCR Reagent Kit was used for real-time PCR in a 7900HT Fast Real-Time PCR machine (Applied Biosystems Inc., Foster City, CA). As a control, PP2A was used to normalize the expression of other genes. Following manufacturer’s instruction (Applied Biosystems Inc., Foster City, CA), the resulting cycle threshold (Ct) values were used to calculate the levels of expression of different genes relative to PP2A . Supplementary Table 1 online describes all the primer sequences used for qRT–PCR assays. Protein extraction and immunoblot analyses The protein extraction from seedlings and immunoblot analyses were performed as described [17] . Briefly, 0.02 g seeds of Col-0 and various mutants were sterilized, plated on MS plates with filter paper and stratified at 4 °C for 4 days. After 3 h of white light treatment for induction of germination, plates were kept in darkness for 4 days at 21 °C. The true dark conditions used here has been previously described [24] . Briefly, 0.02 g of Col-0 seeds were sterilized and plated within 1.5 h in white light. The plates were stratified at 4 °C for 5 days and then exposed to 15 min of FR light (3.2 μmol m −2 s −1 ) before being kept in darkness for four additional days at 21 °C. Total proteins were extracted from 0.2 g tissue of 4-day-old dark-grown seedlings in 800 μl extraction buffer (1 M MOPS pH 7.6, 0.5 M EDTA, pH 8, 50% glycerol, 10% SDS, 40 mM β-mercaptoethanol and 1 × protease inhibitor cocktail (Sigma-Aldrich Co., St Louis, MO, Catalogue (Cat.) No: P9599), 1 mM phenylmethylsulfonyl fluoride (PMSF), 25 mM β- glycerophosphate, 10 mM NaF and 2 mM sodium orthovanadate) with or without different light treatment indicated in individual figures. Samples were boiled immediately for 3 min and centrifuged at 16,000 g for 10 min at room temperature. Thirty-microlitre supernatants of individual samples were loaded on an 8% SDS-polyacrylamide gel electrophoresis (PAGE) gels. The total proteins were blotted onto polyvinylidene difluoride (PVDF) membranes, and probed with native anti-PIF1 (ref. 17 ; 1:5,000 dilutions) and anti-RPT5 (1:1,000 dilutions; Enzo Life Sciences, Farmingdale, NY, cat. no: PW8375-0100) antibodies. For the quantification of the degradation kinetics, we used publicly available ImageJ software to measure band intensities based on at least three biological repeats data. Uncropped western blots for PIF1 levels in Fig. 1 are shown in Supplementary Fig. 11 . The protein extraction from seeds and immunoblot analyses were performed as described [49] . Briefly, 0.02 g seeds of Col-0 and various mutants were sterilized and plated on filter paper in MS plates within 1 h. The plates were exposed to FR light (3.2 μmol m −2 s −1 ) for 15 min before being kept in the dark for 48 h at 21 °C. For red light treatment, the plates were either kept in darkness or exposed to a pulse of 15 μmol m −2 red light pulse and stored in the dark for 1 and 2 h. For far-red light treatment, the seeds were then either kept in darkness or exposed to 5 μmol m −2 s −1 of continuous far-red light for 1 and 3 h. All seed tissues were collected in the dark and ground into powder in liquid nitrogen. For individual sample, total protein was extracted in 50 μl urea extraction buffer (0.1 M phosphate buffer pH 6.8, 0.01 M Tris·Cl, pH 6.8, 48% urea (w/v), 1 mM PMSF, 40 μM bortizomib and 1 × protease inhibitor cocktail (Sigma-Aldrich Co., St Louis, MO, Cat No: P9599). Samples were centrifuged at 16,000 g for 10 min at 4 °C. Supernatants were filtered through Filtration columns (Sigma-Aldrich Co., St Louis, MO, Cat. No: C6866) and boiled for 3 min with 6 × SDS buffer added. Thirty-microlitre supernatants of individual samples were loaded on an 8% SDS–PAGE gels. The total proteins were blotted onto PVDF membranes and probed with native anti-PIF1 (ref. 17 ; 1:5,000 dilutions) and anti-RPT5 (1:1,000 dilutions; Enzo Life Sciences, Farmingdale, NY, Cat. No: PW8375-0100) antibodies. Uncropped western blots for PIF1 levels in Fig. 5 are shown in Supplementary Fig. 12 . Construction of vectors and generation of transgenic plants The TAP-PIF1, TAP-SPA1, Flag-CUL4, TAP-SPA1/PIF1-HA and TAP-PIF1/COP1-HA transgenic plants have been previously described [6] , [7] , [20] , [29] . The PIF1-HA-pGWB14 plasmid was described [7] . For construction of Flag-CUL4/PIF1-HA transgenic lines, the above PIF1-HA-pGWB14 plasmid was transformed into the Flag-CUL4 transgenic background. Homozygous lines were selected from T3 generation with detectable PIF1-HA expression. Co-immunoprecipitation assays The in vivo/in vitro co-immunoprecipitation assays were performed as described [17] . Briefly, 4-day-old dark-grown seedlings were pretreated with 40 μmol bortezomib (LC Laboratories, Woburn, MA) for at least 4 h. Total proteins were extracted from 0.4 g tissue with 800 μl native extraction buffer (100 mM phosphate buffer, pH 7.8, 150 mM NaCl, 0.1% NP40, 1 × protease inhibitor cocktail (Sigma-Aldrich Co., St Louis, MO, Cat. No: P9599), 1 mM PMSF, 40 μM bortezomib, 25 mM β-glycerophosphate, 10 mM sodium fluoride (NaF) and 2 mM Na orthovanadate). After 15 min centrifugation at 16,000 g at 4 °C in darkness, supernatants were incubated with Dynabeads Protein A (Life Technologies Co., Carlsbad, CA, Cat. No: 10002D) bound with either anti-HA antibody (Abcam, Cambridge, MA, Cat. No: ab9110) or anti-MYC antibody (Sigma-Aldrich Co., St Louis, MO, Cat. No: C3956). Twenty-microlitre Dynabeads with 1 μg antibody were used for individual sample. After 2 h incubation in the dark at 4 °C, beads were washed three times with 1 ml extraction buffer with 0.2% NP40. Immunoprecipitated proteins were eluted with 1 × SDS loading buffer and incubated at 65 °C for 5 min. Samples were loaded on a 6.5% SDS–PAGE gel, blotted onto PVDF membranes and probed with antibodies. For PIF1-HA and CUL4-flag interaction, co-IP was carried out using the anti-HA antibody and then probed with anti-flag (Sigma-Aldrich Co., St Louis, MO, Cat. No: F1804, 1:1,000 dilution) and anti-HA antibodies (Covance Co, Princeton, NJ, Cat. No. 16B12, 1:1,000 dilution). For TAP-PIF1 and COP1-HA interaction, co-IP was carried out using the anti-HA antibody and then probed with anti-myc (EMD Millipore, Billerica, MA, Cat. No. OP10, 1:1,000 dilution) and anti-HA (Covance Co, Princeton, NJ, Cat. No. 16B12, 1:1,000 dilution) antibodies. For PIF1-HA and TAP-SPA1 interaction, co-IP was carried out using the anti-HA antibody and then probed with anti-myc (EMD Millipore, Billerica, MA, Cat. No. OP10, 1:1,000 dilution) and anti-HA (Covance Co, Princeton, NJ, Cat. No. 16B12, 1:1,000 dilution) antibodies. Uncropped western blots for bait and prey levels in Fig. 3 are shown in Supplementary Fig. 13 . For in vitro co-immunoprecipitation assay, MBP-COP1 and His-PIF1 were used as described previously [7] , [32] . MBP–SPA1 was expressed from pMAL–SPA1 vector. The full-length open reading frame of SPA1 was PCR amplified using the primers indicated in Supplementary Table 1 . The PCR product and the vector pMAL-p2X (New England Biolabs, Ipswich, MA) were digested with XbaI and SalI restriction enzymes and then ligated to produce pMAL–SPA1 construct. His-PIF1 was incubated with amylose resin in the binding buffer (50 mM Tris-Cl, pH 7.5, 150 mM NaCl, 0.6% Tween 20 and 1 mM DTT) for 1 h. The beads were collected and washed six times with 5 min of rotation each time in the binding buffer. The samples were boiled and analysed by western blot on PVDF membrane. Anti-His antibody (Santa Cruz Biotechnology, Cat. No: SC-803, 1:500 dilutions) was used to detect His-PIF1. Yeast two-hybrid analyses The cloning of the full-length, different truncated forms and mutant versions of PIF1 have been described previously [7] . The full-length and various truncated forms of SPA1 were PCR amplified using the primers listed in Supplementary Table 1 . The PCR product and the vector pJG4.5 (ref. 50 ) were digested with EcoRI and XhoI restriction enzymes, and then ligated to produce AD-SPA1, AD-SPA1-N696, AD-SPA1-N545, AD-SPA1-CC, AD-SPA1-WD40 and AD-SPA1-C509 constructs. All the constructs were verified by restriction enzyme digestion and sequencing. The yeast two-hybrid assays were performed as described previously [50] . Briefly, different combinations of prey and bait constructs were transformed into the yeast strain, EGY48-0 and selected on -His, -Ura, -Trp minimal synthetic medium at 30 °C for 3–4 days. Similar-size yeast colonies were cultured overnight in liquid media supplemented with 2% (w/v) glucose. Aliquots of overnight cultures were transferred to liquid medium supplemented with 2% (w/v) Gal and 1%(w/v) raffinose to induce the expression of prey proteins. The quantitative β-galactosidase assays were carried out with yeast cell extracts using the substrate o -nitrophenyl-β-d-galactopyranoside (4 mg ml −1 , dissolved in Z buffer). The β-galactosidase activity units =1,000 × OD420/( t × V × OD600); where t =elapsed time (in min) of incubation; V =0.1 ml × concentration factor; OD600=Absorbance at 600 nm of 1 ml of yeast cell culture and OD420=Absorbance at 420 nm of 1 ml of supernatant of each of the o -nitrophenyl-β-d-galactopyranoside reactions. Three independent repeats were performed for the β-galactosidase assays and the average values are shown with standard deviation. How to cite this article : Zhu, L. et al . CUL4 forms an E3 ligase with COP1 and SPA to promote light-induced degradation of PIF1. Nat. Commun . 6:7245 doi: 10.1038/ncomms8245 (2015).